Environmental noise exposure degrades normal listening processes To date, the functional and physiological impact on the mature brain of moderate-level environmental noises that do not cause noticeable peripheral deficits remains largely unstudied. Here we show that exposing adult rats to structured noise at a sound pressure level of 65 dB, which is markedly below the broadly accepted safety level standard, results in behavioural impairments and substantially impairs the function of the auditory cortex. The strong deterioration in cortical processing of acoustic inputs is independent of the modulation rates of structured noises. Almost equally strong effects result from 10-h daily versus 24-h daily exposure regimens. These results indicate that there can be substantial negative consequences for the auditory system documented at the cortical level, attributable to environmental exposure to structured noises delivered under conditions that do not directly impact hearing sensitivity. These noises are deemed to be 'safe' and are often present in modern human environments. People are continuously bombarded by environmental noises with highly variable temporal patterns, intensities (but mostly at moderate levels) and exposure schedules in both modern workplace and living environments. It has long been appreciated that persistent loud noises delivered at levels that induce 'permanent threshold shifts' (for example, above 115 dB sound pressure level (SPL)) can damage the inner ear and can induce enduring negative functional changes recordable in the central auditory nervous system that parallel auditory-related perceptual deficits [1] , [2] , [3] , [4] , [5] , [6] , [7] . Possibly, because the exposure to moderately loud noises does not affect hearing per se , the functional and physiological impact of exposure to non-damaging sounds (below about 85 dB SPL), especially on the mature brain, remains largely unstudied. That is perhaps surprising, given the fact that industrial workers are required to use 'ear protecting' sound attenuation devices that bring sound pressure levels 'safely' down into this loudness range. The functional development of the auditory system is substantially influenced by acoustic inputs during the early stages of life when the system is most susceptible to alteration by acoustic experience. For example, passive exposure of developing animals to specific sounds (for example, tone pips or structured noises) during the critical period of cortical development induces lasting changes in neuronal processing and the tonotopic map in the primary auditory cortex (A1) [8] , [9] , [10] , [11] , [12] , [13] . Such 'passive' exposure during adulthood has generally been considered to have little effect; acoustic inputs, in conjunction with behavioural training [14] , [15] , [16] , [17] , or with stimulation of the basal forebrain system [18] , [19] or vagus nerve [20] , [21] , have been argued to be necessary to induce persistent plastic changes in the mature brain. A few recent studies have challenged this view by showing that housing adult animals in the presence of moderately loud broad-spectrum sounds (~65–70 dB SPL) also results in large-scale cortical changes in animals in which peripheral hearing and hearing thresholds seem to be unaffected [22] , [23] . These studies indicate that there may be potentially destructive consequences induced by environmental noise exposure, even when sounds are limited to the lower intensity levels that are presently considered to be harmless [24] . In this study, 3-month-old rats were exposed to structured noises delivered at 65 dB SPL for a 2-month period. This modulated broad-spectrum noise exposure more realistically models the noise environments encountered in the industrial workplace and other modern acoustic settings. As each modulatory event results in the broad, correlated excitation of neurons across all of A1, temporally modulated noise stimuli might be expected to have a different and more strongly disorganizing impact than the continuous white noises applied in an earlier study [23] . Indeed, significant behavioural impairments and negative cortical changes in temporal and spectral sound processing, as well as parallel chemical and physical changes, were induced in these structured noise-exposed (NE) adult rats. Because human speech and language abilities require the refined spectro-temporal processing of acoustic inputs, our data indicate a probable risk, resulting from long-term moderate-level noise exposure, for degraded auditory and language-related reception and cognitive abilities that would apply for individuals of all ages. Behavioural performance We first examined the behavioural performance of NE versus age-matched control rats by using temporal rate discrimination tasks ( Fig. 1a ). This behavioural evaluation of possible consequences of structured noise exposure consisted of a procedural-learning phase followed by a perceptual-testing phase. In that first experimental phase, rats were trained to discriminate between pulse trains presented at 6.3 pulses per second (p.p.s.) (the 'non-target') and 20 p.p.s. (the 'target'). The detection of this large difference in temporal rate for presented pulse trains (that is, 6.3 p.p.s. versus 20 p.p.s.) was perceptually unchallenging; both NE and control rats learned the task after several days of training. As illustrated in Fig. 1b , which shows the average performance scores across training blocks at the seventh day (that is, the last day of the procedural-learning phase), both rat groups quickly reached a steady performance score on the third training block. However, the average performance score recorded for NE rats ( n =9) was lower than for control rats ( n =12) at every block ( P <0.05–0.001, t -test). 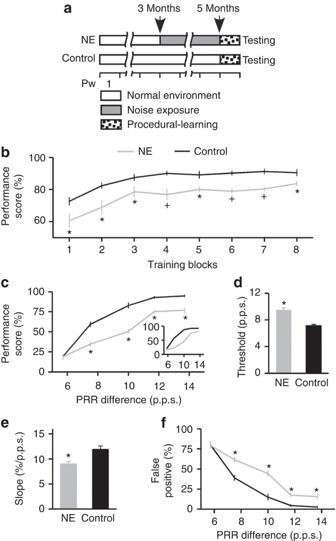Figure 1: Behavioural performance on the temporal rate discrimination task. (a) Experimental timeline. Pw, postnatal weeks. (b) Discrimination performance of NEK (n=9) and control (n=12) rats across training blocks at the seventh training day (that is, the last day of the procedural-learning phase), when the animals were trained to discriminate a pulse train of 6.3 pulses per second (p.p.s.; that is, non-target) from that of 20 p.p.s. (target). Error bars represent s.e.m. *P<0.05, +P<0.001,t-test. (c) Average psychometric curves obtained from NE rats at the eighth training day (that is, 1 week after the end of noise exposure) and from age-matched control rats. Inset shows examples of the psychometric curves. PRR, pulse repetition rate. *P<0.0001,t-test. (d) Comparison of discrimination thresholds for NE and control rats. *P<0.0001,t-test. (e) Average slopes of the psychometric curves for NE and control rats. The slope of each psychometric curve was calculated at its steepest portion (difference in performance score for changing the PRR difference from 5.7 to 11.7 p.p.s.). *P<0.005,t-test. (f) The false positive ratio as a function of PRR difference for NE and control rats. *P<0.001,t-test. Figure 1: Behavioural performance on the temporal rate discrimination task. ( a ) Experimental timeline. Pw, postnatal weeks. ( b ) Discrimination performance of NEK ( n =9) and control ( n =12) rats across training blocks at the seventh training day (that is, the last day of the procedural-learning phase), when the animals were trained to discriminate a pulse train of 6.3 pulses per second (p.p.s. ; that is, non-target) from that of 20 p.p.s. (target). Error bars represent s.e.m. * P <0.05, + P <0.001, t -test. ( c ) Average psychometric curves obtained from NE rats at the eighth training day (that is, 1 week after the end of noise exposure) and from age-matched control rats. Inset shows examples of the psychometric curves. PRR, pulse repetition rate. * P <0.0001, t -test. ( d ) Comparison of discrimination thresholds for NE and control rats. * P <0.0001, t -test. ( e ) Average slopes of the psychometric curves for NE and control rats. The slope of each psychometric curve was calculated at its steepest portion (difference in performance score for changing the PRR difference from 5.7 to 11.7 p.p.s.). * P <0.005, t -test. ( f ) The false positive ratio as a function of PRR difference for NE and control rats. * P <0.001, t -test. Full size image On the eighth day, all animals with identical procedural-learning histories underwent a second perceptual-testing phase in which the non-target at each trial was randomly chosen from pulse trains of various repetition rates (6.3, 8.3, 10, 12.5, or 14.3 p.p.s.). A psychometric curve was then constructed to define the temporal rate discrimination ability of each animal. As shown in Fig. 1c , whereas the performance scores for rats of both groups increased as the rate difference between target and non-target increased, values at rate differences larger than 5.7 p.p.s. were significantly lower for NE than for control rats (all P <0.0001, t -test). That difference was supported by an analysis of the discrimination threshold, defined as the rate difference corresponding to a 50% performance score on the psychometric curve. That threshold was significantly higher in NE rats than in control rats ( Fig. 1d ; P <0.0001, t -test). The slope of psychometric curve for NE rats, however, was smaller than for control rats ( Fig. 1e ; P <0.005, t -test). Additionally, the false positive ratios for both NE and control rats decreased as the rate difference between target and non-target increased ( Fig. 1f ). Those changes were less for NE than for control rats (all P <0.001, t -test). The results showed that a 2-month-long exposure to moderate-level structured noises significantly degraded these adult animals' abilities to discriminate between sound stimulus rates. These recorded post-exposure effects persisted for at least 6 weeks after the end of noise exposure ( Supplementary Fig. S1 ). ABR thresholds and cortical responses Auditory brainstem response (ABR) measurement and cortical recording were conducted on NE rats 1 week after they were returned to a normal sound environment. Data were then compared with those recorded in age-matched control rats ( Fig. 2a ). 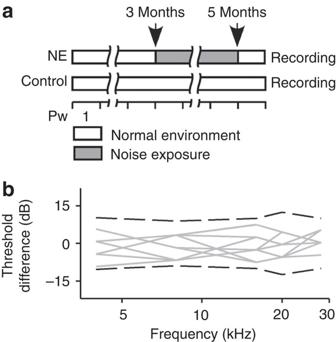Figure 2: ABR thresholds. (a) Experimental timeline. Pw, postnatal weeks. (b) ABR thresholds obtained from NE rats (n=8) relative to normative ABR thresholds of control rats (n=12). Positive values indicate higher ABR thresholds compared with controls. Dashed lines, range of normative ABR thresholds (±2 s.d.). Figure 2: ABR thresholds. ( a ) Experimental timeline. Pw, postnatal weeks. ( b ) ABR thresholds obtained from NE rats ( n =8) relative to normative ABR thresholds of control rats ( n =12). Positive values indicate higher ABR thresholds compared with controls. Dashed lines, range of normative ABR thresholds (±2 s.d.). Full size image As shown in Fig. 2b , all ABR data recorded from NE rats were within the normal±2 s.d. boundaries. Statistical analysis showed no significant threshold differences between NE ( n =8) and control ( n =12) rats at any frequency determined (all P >0.39, t -test). Cortical responses were also recorded from 322 sites in 7 NE rats and from 369 sites in 8 age-matched control rats (see Fig. 2a for the experimental line). Response thresholds and latencies recorded at cortical sites in NE rats (22.1±0.7 dB SPL and 11.5±0.1 ms; mean±s.e.m.) did not differ from those recorded in control rats (20.6±0.7 dB SPL and 11.4±0.1 ms; both P >0.1, t -test). The frequency selectivity was first evaluated for each cortical site by constructing the tuning curve using tone pips with random frequencies and intensities ( Fig. 3a ). The tuning curve bandwidths measured 20 dB above threshold (BW20 s) were larger for NE than for control rats ( Fig. 3b ; P <0.01–0.00001, t -test), indicating that the frequency response selectivity was significantly and systematically degraded by noise exposure. We further examined the similarity of the tuning curves recorded from neighbouring cortical neurons (that is, overlap index) to evaluate the extent of spatial activation overlap in the A1 ( Fig. 3c ). As expected, the average overlap index systematically changed as a function of distance between recording sites for both rat groups. The index of NE rats, however, was significantly larger than that of control rats for distances smaller than 1.2 mm ( P <0.001–0.00001, t -test). 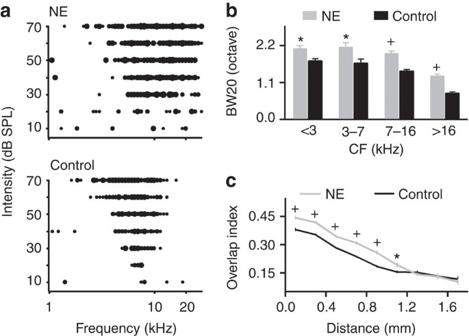Figure 3: Cortical frequency selectivity. (a) Representative examples of tuning curves obtained from NE and control rats. (b), Average receptive field bandwidths at 20 dB above threshold (BW20s) for all recording sites in NE (recording sites=322) and control (recording sites=369) rats, for each of four CF ranges. Bin size=1.2 octave. Error bars represent s.e.m. *P<0.01,+P<0.00001,t-test. (c) Average tuning curve overlap index as a function of distance between recording sites for NE and control rats. *P<0.001, +P<0.00001,t-test. Figure 3: Cortical frequency selectivity. ( a ) Representative examples of tuning curves obtained from NE and control rats. ( b ), Average receptive field bandwidths at 20 dB above threshold (BW20s) for all recording sites in NE (recording sites=322) and control (recording sites=369) rats, for each of four CF ranges. Bin size=1.2 octave. Error bars represent s.e.m. * P <0.01, + P <0.00001, t -test. ( c ) Average tuning curve overlap index as a function of distance between recording sites for NE and control rats. * P <0.001, + P <0.00001, t -test. Full size image When tested with characteristic frequency (CF) tone pulses delivered at variable rates, most cortical neurons in control rats followed repeated identical stimuli at and below rates of 10 p.p.s., with each brief tone evoking about the same number of spikes as did the first tone in a stimulus train. Numbers of responses per tone then fell off rapidly at still higher repetition rates. By contrast, most neurons in NE rats followed stimuli at or below repetition rates of only about 7 p.p.s. ( Fig. 4a , left versus right). These effects were further documented by deriving repetition rate transfer functions (RRTFs) recorded for neurons at each cortical site ( Fig. 4a , insets). Although the average RRTFs took a low-pass form in both rat groups, values at high temporal rates (>7 p.p.s.) for NE rats were significantly lower than in control rats ( Fig. 4b ; recording sites=316 for NE rats and 368 for control rats; P <0.05–0.0005, t -test). 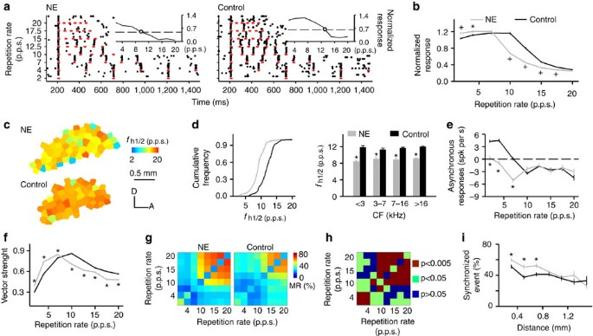Figure 4: Cortical temporal responses. (a) Dot-raster plot examples of cortical responses to pulse trains of different repetition rates recorded from NE and control rats. Red lines indicate pulse durations. Inset shows the RRTF for each raster plot example. Unfilled circle and dashed line showfh1/2and 50% of the maximal normalized response for each RRTF, respectively. (b) Average RRTFs for all recordings obtained from NE (recording sites=316) and control (recording sites=368) rats. Error bars represent s.e.m. *P<0.05, +P<0.0005,t-test. (c) Representative auditory corticalfh1/2maps for NE and control rats. The colour of each polygon indicates thefh1/2recorded at that site. D, dorsal; A, anterior. (d) Cumulative frequency histograms (left) showing a significant leftward shift of thefh1/2distribution for NE rats compared with control rats (Kolmogorov–Smirnov test,P<0.0001), and averagefh1/2s (right) for all recording sites in both rat groups, for each of four CF ranges. Bin size=1.2 octaves. *P<0.0005,t-test. (e) Average asynchronous response rates measured at different pulse repetition rates for NE and control rats. *P<0.00001,t-test. (f) Average vector strengths measured at different pulse repetition rates for NE and control rats. *P<0.0005,t-test. (g) Average MR obtained using the Van Rossum spike train distance metric for all combination of repetition rates, for NE and control rats. (h) Results oft-test for comparisons of MR between NE and control rats. (i) Percentage of synchronized spontaneous discharge as a function of distance between two cortical recording sites. *P<0.008,t-test. Figure 4: Cortical temporal responses. ( a ) Dot-raster plot examples of cortical responses to pulse trains of different repetition rates recorded from NE and control rats. Red lines indicate pulse durations. Inset shows the RRTF for each raster plot example. Unfilled circle and dashed line show f h1/2 and 50% of the maximal normalized response for each RRTF, respectively. ( b ) Average RRTFs for all recordings obtained from NE (recording sites=316) and control (recording sites=368) rats. Error bars represent s.e.m. * P <0.05, + P <0.0005, t -test. ( c ) Representative auditory cortical f h1/2 maps for NE and control rats. The colour of each polygon indicates the f h1/2 recorded at that site. D, dorsal; A, anterior. ( d ) Cumulative frequency histograms (left) showing a significant leftward shift of the f h1/2 distribution for NE rats compared with control rats (Kolmogorov–Smirnov test, P <0.0001), and average f h1/2 s (right) for all recording sites in both rat groups, for each of four CF ranges. Bin size=1.2 octaves. * P <0.0005, t -test. ( e ) Average asynchronous response rates measured at different pulse repetition rates for NE and control rats. * P <0.00001, t -test. ( f ) Average vector strengths measured at different pulse repetition rates for NE and control rats. * P <0.0005, t -test. ( g ) Average MR obtained using the Van Rossum spike train distance metric for all combination of repetition rates, for NE and control rats. ( h ) Results of t -test for comparisons of MR between NE and control rats. ( i ) Percentage of synchronized spontaneous discharge as a function of distance between two cortical recording sites. * P <0.008, t -test. Full size image We quantified the cortical capacity for processing high-rate stimuli by determining the highest modulation rate at which RRTF was at half-maximum (that is, f h1/2 ; Fig. 4a , insets). As shown in Fig. 4c , where we illustrate f h1/2 maps for representative NE and control rats, the f h1/2 s obtained at most cortical sites in NE rats were lower than in control rats. A quantitative comparison of the distribution for all f h1/2 s obtained from both rat groups is shown in Fig. 4d (left). A significant leftward shift of the f h1/2 distribution for NE rats compared with control rats ( P <0.0001, Kolmogorov–Smirnov test) confirmed a degraded rate-following ability induced by this chronic noise exposure. Interestingly, this degradation was recorded for neurons extending across all CF ranges ( Fig. 4d , right; all P <0.0005, t -test). Earlier studies have shown that the rate-following ability of cortical neurons is proportionally related to the degree of post-stimulus suppression [25] . Here we quantified the asynchronous response, defined as the mean firing rate outside the phase-locking windows minus the spontaneous firing rate for both NE and control rats, to evaluate the post-stimulus suppression ( Fig. 4e ). Asynchronous responses were weaker at low temporal rates in NE rats, indicating stronger and/or longer post-stimulus suppression compared with control rats (all P <0.00001, t -test). To characterize the temporal fidelity of cortical responses, we calculated vector strengths, which quantify the degree of phase locking of neural responses to repetitive stimuli. As shown in Fig. 4f , average vector strengths as a function of temporal rates shifted leftward and peaked at lower rates in NE compared with control rats (peak at 7 p.p.s. in NE rats versus 10 p.p.s. in control rats). In addition, vector strengths of neurons in NE rats were smaller at high repetition rates (that is, 10–20 p.p.s.) but greater at low rates (that is, 2–7 p.p.s. ; all P <0.0005, t -test). We further examined the reliability of cortical responses to repetitive stimuli by calculating the misclassification rate (MR) for every possible combination of pulse trains used to construct the RRTFs ( Fig. 4g ). That measurement, obtained using the Van Rossum spike train distance metric [26] , quantifies the similarity between spike trains recorded, using different pulse trains, or the difference between spike trains recorded, using identical pulse trains. Larger MR values indicate more confusable and unreliable spike trains representing temporal structure in acoustic inputs. We found that the average MRs for combinations of dissimilar high pulse rates (10–20 p.p.s.) were significantly larger in NE versus control rats ( Fig. 4g and h ). The average numbers of 'misrepresentations' of identical stimuli were greater in NE rats, markedly at lower pulse rates (that is, 2 p.p.s. versus 2 p.p.s., or 4 p.p.s. versus 4 p.p.s. ; Fig. 4h ). To assess horizontal cortical network connectivity, we calculated correlation coefficients for neuron pairs separated by variable distances by simultaneously recording their spike discharges during spontaneous activity periods. Correlation coefficients quantify the degree of cortical horizontal connectivity, with higher values representing stronger horizontal connections. We considered all spikes that occurred in two recording channels, within 10 ms of one another, to be synchronized events. The average correlation coefficient between −10 and 10 ms lags was 31% larger for NE than for control rats ( P <0.00001, t -test). The degree of synchronization for simultaneously recorded spontaneous discharges, expressed as a percentage of synchronized events, significantly decreased as a function of inter-electrode distances in both rat groups ( Fig. 4i ; both P <0.0001, ANOVA). However, values were higher at electrode separations less than 1.3 mm in NE than in control rats ( P <0.008 at electrode separations of 0.3, 0.5 and 0.7 mm; t -test). In accordance with behavioural data, cortical changes in temporal processing, induced by noises, endured for at least 6 weeks after the end of noise exposure ( Supplementary Fig. S2 ). Passive sound exposure-driven plasticity in A1 To determine whether or not structured noise exposure restores passive sound exposure-driven plasticity in the frequency representation domain in mature cortices, a subset of NE rats were exposed to pulsed 7-kHz tones for 1 week, beginning at the end of their noise exposure epoch (these rats were defined as NE plus tone-exposed rats (TE), that is, NE+TE rats in Fig. 5a ). As an additional control, another group of age-matched control rats were also exposed to pulsed 7-kHz tones over the same epoch (these rats were defined as tone-exposed rats, that is, TE rats in Fig. 5a ). To quantitatively characterize the effects of pulsed tone exposure on A1-frequency representation, percentages of A1 areas representing different frequency ranges were averaged within the same experimental group and differences between exposed and control animals plotted. As shown in Fig. 5b , the percentages of A1 areas representing each frequency range for NE+TE ( n =6) and TE ( n =4) rats were comparable to that in control ( n =8) rats (all P >0.3, ANOVA). This result, in contrast to our recent report that applied continuous unstructured noises [23] , showed that structured noise exposure did not result in the re-opening of an epoch of critical period-like plasticity. 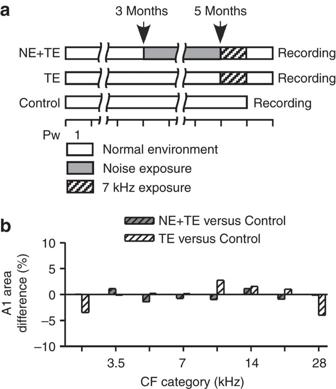Figure 5: Structured noise exposure does not restore the passive sound exposure-driven plasticity. (a) The experimental timeline for NE plus tone-exposed (NE+TE), tone-exposed (TE), and control rats. Pw, postnatal weeks. (b) Differences in percentages of A1 areas tuned to different frequency ranges for NE+TE (n=6) or TE (n=4) versus control (n=8) rats. Figure 5: Structured noise exposure does not restore the passive sound exposure-driven plasticity. ( a ) The experimental timeline for NE plus tone-exposed (NE+TE), tone-exposed (TE), and control rats. Pw, postnatal weeks. ( b ) Differences in percentages of A1 areas tuned to different frequency ranges for NE+TE ( n =6) or TE ( n =4) versus control ( n =8) rats. Full size image Effects of exposure to noises presented at different temporal rates All data described above were recorded from NE rats that were exposed to pulse trains with repetition rates that varied over a significant frequency range ( Fig. 6a , top). To investigate how temporal rates of environmental noises might direct exposure-induced cortical changes, additional groups of adult rats were exposed to 1-s pulse trains delivered at fixed repetition rates of either 5 p.p.s. ( Fig. 6a , middle) or 15 p.p.s. ( Fig. 6a , bottom), again for 2 months (24 h per day). Cortical RRTFs were then constructed and compared with those obtained from rats exposed to noises of mixed rates as described earlier, and again, with those from age-matched control rats. Statistical analysis showed that RRTFs and f h1/2 s recorded from different NE groups were comparable ( Fig. 6b and c ; P >0.05 for all comparisons, ANOVA with post-hoc Student–Newman–Keuls test) but were significantly different from that of control rats ( P <0.05–0.001 for all comparisons, except for RRTF values at 7 p.p.s., and for NE-15 p.p.s. and NE versus control rats at 20 p.p.s., ANOVA with post-hoc Student-Newman-Keuls test). These results showed, to our surprise, that post-exposure cortical changes were independent of the modulatory rates of structured noises that animals were exposed to. As expected, cortical response thresholds and latencies recorded from different rat groups did not significantly differ ( Fig. 6d and e ; both P >0.16, ANOVA). 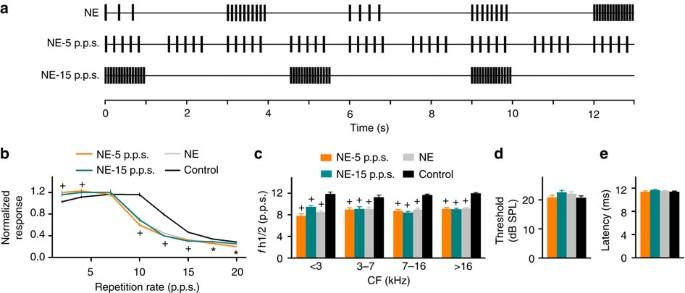Figure 6: Effects of temporal rates of noises on cortical responses. (a), Schematic of the stimuli used in the different noise-exposure conditions. For the first condition, 1-s pulse train with repetition rates of 3, 4, 8, 10, 12, 15 or 18 p.p.s. was randomly presented (top). For the other two conditions, the repetition rate of 1-s pulse train was either set at 5 p.p.s. (middle) or 15 p.p.s. (bottom). These pulse trains were presented once every 3, 1.5, or 4.5 s such that the total acoustic energy of noise bursts received by rats of all three groups was approximately equal during the 2-month's exposure. (b,c), Average RRTFs (b) andfh1/2s (c) obtained from different NE groups (recording sites=180 for NE-5 p.p.s. rats, 230 for NE-15 p.p.s. rats, and 316 for NE rats, respectively), illustrated with that of age-matched control rats (recording sites=368). Error bars represent s.e.m. *P<0.05,+P<0.001 compared with controls, ANOVA withpost-hocStudent-Newman-Keuls test. (d,e), Response thresholds (d) and latencies (e) recorded from different NE groups, illustrated with control rats. Figure 6: Effects of temporal rates of noises on cortical responses. ( a ), Schematic of the stimuli used in the different noise-exposure conditions. For the first condition, 1-s pulse train with repetition rates of 3, 4, 8, 10, 12, 15 or 18 p.p.s. was randomly presented (top). For the other two conditions, the repetition rate of 1-s pulse train was either set at 5 p.p.s. (middle) or 15 p.p.s. (bottom). These pulse trains were presented once every 3, 1.5, or 4.5 s such that the total acoustic energy of noise bursts received by rats of all three groups was approximately equal during the 2-month's exposure. ( b,c ), Average RRTFs ( b ) and f h1/2 s ( c ) obtained from different NE groups (recording sites=180 for NE-5 p.p.s. rats, 230 for NE-15 p.p.s. rats, and 316 for NE rats, respectively), illustrated with that of age-matched control rats (recording sites=368). Error bars represent s.e.m. * P <0.05, + P <0.001 compared with controls, ANOVA with post-hoc Student-Newman-Keuls test. ( d,e ), Response thresholds ( d ) and latencies ( e ) recorded from different NE groups, illustrated with control rats. Full size image Effects of intermittent noise exposure To investigate the effects of intermittent noise exposure on cortical temporal responses, 5 additional adult rats were exposed to noise stimuli (as shown at the top of Fig. 6a ) for 10 h per day followed by 14 h in the quiet, simulating a noisy-work/quiet-living environment. These passive exposure epochs again extended over a 2-month period beginning at 3 months of age. As shown in Fig. 7a , average RRTFs at higher temporal rates (>7 p.p.s.) were significantly smaller for these NE than for control rats ( P <0.005–0.00001, t -test). And again, average f h1/2 s in NE rats were lower than that of control rats at every CF range ( Fig. 7b ; P <0.05–0.00001, t -test). 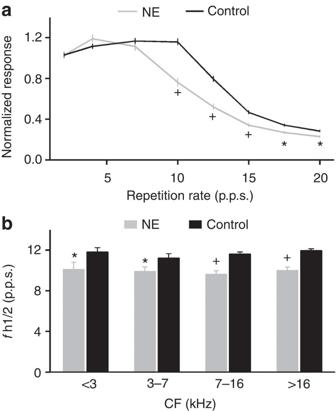Figure 7: Effects of intermittent noise exposure on cortical temporal responses. (a) Average RRTFs for all recordings obtained from NE (recording sites=219) and control (recording sites=368) rats. NE rats were exposed to noise stimuli (as shown at the top ofFig. 6a) for 10 h per day followed by 14 h in the quiet, simulating a noisy-work/quiet-living environment. Error bars represent s.e.m. *P<0.005, +P<0.00001,t-test. (b), Averagefh1/2s for all recording sites in NE and control rats for each of four CF ranges. *P<0.05, +P<0.00001,t-test. Figure 7: Effects of intermittent noise exposure on cortical temporal responses. ( a ) Average RRTFs for all recordings obtained from NE (recording sites=219) and control (recording sites=368) rats. NE rats were exposed to noise stimuli (as shown at the top of Fig. 6a ) for 10 h per day followed by 14 h in the quiet, simulating a noisy-work/quiet-living environment. Error bars represent s.e.m. * P <0.005, + P <0.00001, t -test. ( b ), Average f h1/2 s for all recording sites in NE and control rats for each of four CF ranges. * P <0.05, + P <0.00001, t -test. Full size image Physical indices of neurological changes To begin to determine how physical changes in cortical networks might contribute to these noise-induced changes in cortical temporal processing, we first quantified the expression levels of parvalbumin (PV), by using immunohistochemical methods. We found significant decreases in the numbers of PV-immunostained (PV+) neurons across cortical layers II–VI in A1 in NE compared with control rats ( Fig. 8a versus b, left; and Fig. 8c , all P <0.00001, t -test). Percentage decreases were 32.7, 43.3, 37.2 and 30.1% for layers II–III, IV, V, and VI, respectively. Reduced dendritic PV immunoreactivity was also noted in NE rats compared with control rats ( Fig. 8d versus e, arrows). 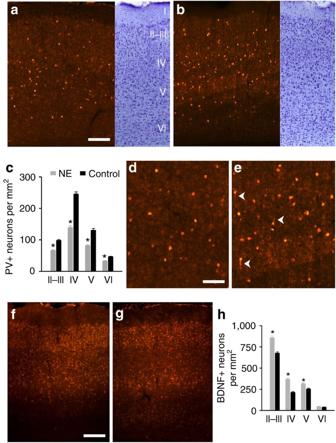Figure 8: Expression levels of cortical PV and BDNF. (a,b), Photomicrographs of PV-immunostained (PV+, left) and Nissl-stained (right) cortical sections for NE (a) and control (b) rats. NE rats were exposed to noise stimuli shown at the top ofFig. 6afor 2 months (24 h per day) beginning at 3 months of age. Cortical layers are indicated in Nissl-stained sections. Scale bar, 200 μm. (c), Average PV+ neuron counts for NE (12 hemispheres) and control (12 hemispheres) rats. Error bars represent s.e.m. *P<0.00001,t-test. (d,e), Higher magnification photomicrographs showing the reduced dendritic PV immunoreactivity in NE (d) compared with control (e) rats (arrows). Scale bar presents 100 μm. (f,g), Photomicrographs of BDNF-immunostained (BDNF+) cortical sections for NE (f) and control (g) rats. Scale bar, 200 μm. (h) Average BDNF+ neuron counts for NE (16 hemispheres) and control (16 hemispheres) rats. *P<0.0005,t-test. Figure 8: Expression levels of cortical PV and BDNF. ( a,b ), Photomicrographs of PV-immunostained (PV+, left) and Nissl-stained (right) cortical sections for NE ( a ) and control ( b ) rats. NE rats were exposed to noise stimuli shown at the top of Fig. 6a for 2 months (24 h per day) beginning at 3 months of age. Cortical layers are indicated in Nissl-stained sections. Scale bar, 200 μm. ( c ), Average PV+ neuron counts for NE (12 hemispheres) and control (12 hemispheres) rats. Error bars represent s.e.m. * P <0.00001, t -test. ( d,e ), Higher magnification photomicrographs showing the reduced dendritic PV immunoreactivity in NE ( d ) compared with control ( e ) rats (arrows). Scale bar presents 100 μm. ( f,g ), Photomicrographs of BDNF-immunostained (BDNF+) cortical sections for NE ( f ) and control ( g ) rats. Scale bar, 200 μm. ( h ) Average BDNF+ neuron counts for NE (16 hemispheres) and control (16 hemispheres) rats. * P <0.0005, t -test. Full size image We also applied the same approach to measure the expression levels of brain-derived neurotrophic factor (BDNF). BDNF is an enabler of cortical growth and plasticity, and is linked in its actions to the expression of inhibitory neurons [23] , [27] , [28] . We found that the numbers of BDNF-immunostained (BDNF+) neurons in layers II–V were significantly increased for NE compared with control rats ( Fig. 8f versus g; and Fig. 8h ; all P <0.0005, t -test). That increase of BDNF+ neurons was more pronounced in cortical layer IV (73.1%) than in layers II–III or V (27% and 23.9%, respectively). We found that mature rats experiencing structured noises for 2 months exhibited significant sound rate discrimination behavioural deficits. In parallel, there was large-scale degradation in cortical temporal processing, manifested by poorer neuronal spike rate-following ability and by decreased response synchronization and response reliability to higher-rate modulated sound stimuli. That degraded response synchronization was recorded even while, paradoxically, a stronger correlation of spontaneous discharges indicated that stronger-than-normal positive coupling had been induced by exposure to structured noises in local networks. These negative changes endured without significant self-correction for at least 6 weeks after the end of noise exposure. A decreased PV expression level and an increased BDNF expression level were also recorded in A1 as a result of noise exposure. However, no measurable changes in ABR thresholds and cortical thresholds and response latencies were found. This study thus provides evidence that chronic exposure to moderate level of structured noises during adulthood can significantly and persistently impair central auditory processing and auditory-related perceptual abilities. It has been compellingly argued that decreased cortical response selectivity and reliability degrade the neurological encoding of the details of acoustic inputs, and thereby impairs auditory-related perceptual abilities [12] , [13] . Consistent with that conclusion, cortical deficits plausibly account for the reduced behavioural performance abilities seen in NE rats. However, we cannot exclude the possibility that sub-cortical sources also contribute to the observed post-exposure behavioural deficits as experience-dependent plasticity has been reported in the inferior calicles of mice and rats [29] , [30] . The discrimination task applied in this study requires animals to identify a fixed, remembered target auditory stimulus from a set of distracter auditory stimuli. This task, therefore, has significant memory and discrimination components. We also recorded significant post-exposure changes in the expression levels of cortical PV and BDNF, two contributors to the regulation of adult cortical plasticity [23] , [27] , [28] , [31] , [32] . Cortical PV+ neurons represent a major part of the GABAergic population in the auditory cortex [33] , and have been shown to modulate cortical response synchronization and firing-timing precision [34] . The relatively sluggish cortical temporal responses, following noise exposure observed here, are very similar to those resulting from reduced cortical GABAergic inhibitions [35] . The decreased PV expression as has been recorded in NE rats, in this study, would certainly be expected to contribute to degradation in cortical temporal responses, and in the representations of temporal features in complex acoustic inputs like aural speech. In addition, an interaction between cortical BDNF and GABAergic inhibition has recently been shown to regulate ocular dominance plasticity in adult visual cortex [27] , [28] . In that system, investigators have recorded higher cortical BDNF levels and lower GABAergic levels, when enriched environments restored ocular dominance plasticity in the rat visual cortex [27] . How these interdependent molecular changes might contribute to the regulation of noise-induced plasticity in the adult auditory cortex remains to be studied. Although chronic exposure of adult rats to structured noises drives negative cortical changes, it does not reinstate critical period-like plasticity in their already mature cortices, in contradistinction to the results of a recent study that exposed post-critical-period rats to continuous, unstructured ('white') noises [23] . In the present study, cortical BDNF expression levels were enhanced following structured noise exposure; with continuous noise exposures, the BDNF levels were significantly lowered. It has been argued that BDNF expression is controlled by local response correlation reflected, for example, in the correlation of spontaneous activity within local cortical networks [36] . That is consistent with these induced changes because BDNF upregulation is here paralleled by stronger-than-normal local network coupling, presumably generated by the modulated spectrally non-selective inputs that are broadly engaging A1. Continuous noise exposure, however, has the opposite effect: a downregulation of BDNF is paralleled by a decrease in local cortical network coupling. Last, animals exposed to non-structured noises recovered normal cortical functionality within several weeks following the cessation of sound exposure. Animals in the current study did not recover. Many weeks after sound exposure, the induced A1 distortions were virtually identical to those recorded immediately after the cessation of sound exposure. More recently, lasting changes in the auditory cortex (that is, suppression of spikes and local field potentials) have also been reported in adult cats that were chronically exposed to pulsatile band-limited noises of ~70 dB SPL [22] 22. Taken together, these findings show that chronic exposure to acoustic stimuli during adulthood, even absent behavioural relevance for that sound exposure, can induce substantial plastic changes documented at the cortical level [22] , [23] , [37] . It should be noted that virtually identical post-exposure changes in cortical temporal responses were recorded in rats that were exposed to structured noises delivered at consistently high or consistently low modulation rates, or at rates that were randomly varied stimulus by stimulus. This suggests that induced changes are dependent on the delivery of a heavy schedule of sharp-onset transient stimulus events, independent of specific modulation rates. Earlier studies have shown that acoustic stimuli paired with perceptual training or electrical stimulation of the nucleus basalis, also induces significant cortical plasticity in the temporal domain in the mature brain [13] , [19] , [25] . These cortical changes, however, are highly specific to the temporal structures and schedules of the applied acoustic stimuli. For example, cortical rate-following abilities were enhanced for rats trained to find a target location using the temporal rate of repetitive stimuli as the only cue, because the target location was always correlated with high rates in the task [25] . The temporal following rate of cortical neurons could also be increased or decreased, depending on the modulation rate of acoustic input paired with NB stimulation [19] . These learning phenomena (that is, refs 19 , 25 ) obviously engage different processes from those engaged by noise exposure outside a behavioural context, as in the present experiments. The present study also illustrates potentially destructive consequences of even moderate-level noise exposure for neurological operations in listening and aural language of older children and adults. Noise-exposure safety regulations have long been based on noise intensity levels that do not demonstrably induce permanent damage to the inner ear [38] , [39] . Although some studies have clearly revealed an impact of moderate-level noise pollution on cognitive development [40] , [41] , the usual explanations for the origins of such effects have invoked stress-related mechanisms. Here we show that chronic exposure to moderate-level noises during adulthood impairs behavioural and neuronal discrimination of sounds in the temporal domain, but with no peripheral deficits. We cannot entirely rule out a possible contribution to these changes from noise-induced stress. At the same time, changes in A1 influenced the representations of the spectral and temporal features of acoustic stimuli. We also carefully monitored sleep and activity patterns, recording no differences between sound-exposed and control animal cohorts. To the extent to which a 'stress response' contributes to these effects, it would presumably also contribute to responses in human populations similarly exposed to moderate-level noises. Qualitatively similar post-exposure effects were also documented even when exposure was limited to 10 h per day, an exposure regimen that better models a noisy-work/quiet-living environment. Noise levels driving these large-scale behavioural and cortical changes in the rat model are of the intensity of a room air conditioner fan. Long-term daily exposure to such noises is commonplace in modern home and workplace environments [42] , [43] . It is likely that less continuous and even milder forms of noise exposure than were applied here could be expected to significantly impair perceptual and cognitive development in children, and to slowly degrade cognitive performance abilities in adults but without any noticeable effect on the hearing threshold. Our results argue strongly for the importance of more completely defining these possible hitherto-unappreciated hazards of noise pollution that cannot be detected with the standard audiogram, in modern human environments. All experimental procedures were approved by the Animal Care and Use Committees at the East China Normal University and the University of California, San Francisco. Sound exposure Female Sprague-Dawley rats, aged 3 months, were randomly divided into two groups: NE and control rats. The NE rats in a cage (35cm×22cm×20 cm, length×width×height) were placed in a sound-shielded test chamber for noise exposure (24 h per day unless specified otherwise). A 1-s pulse train containing 50-ms noise bursts (65 dB SPL; 5-ms ramps) was presented once every 3 s. The repetition rate of each pulse train was randomly set at 3, 4, 8, 10, 12, 15, or 18 p.p.s. ( Fig. 6a , top). The energy for structured noises was essentially flat across a broad frequency spectrum (0.8–30 kHz). Rats were given free access to food and water under an 8-h light/16-h dark cycle. The control rats were reared under same conditions but without exposure to noises. The researcher was held blind to the group identity of the animals. The weights and activities of exposed rats were continuously monitored, and compared with age-matched control rats. The weights of the exposed rats were comparable to control rats and there were no abnormalities in the behaviour of exposed rats. Behavioural testing The behavioural examination consisted of two phases: a procedural-learning phase and a perceptual-testing phase. In the first phase, the rats were trained to discriminate a 520-ms pulse train of 4 noise bursts (that is, non-target; corresponding to temporal rate of 6.3 p.p.s.) from an 11-burst train of the same duration (target; corresponding to temporal rate of 20 p.p.s.). During the perceptual-testing phase, the temporal rate discrimination ability was tested by randomly delivering 520-ms non-target pulse trains with pulse rates of 6.3 p.p.s., 8.3 p.p.s., 10 p.p.s., 12.5 p.p.s., or 14.3 p.p.s., respectively. Training was conducted in an acoustically transparent operant training chamber (20 cm×20 cm×18 cm, length×width×height) enclosed within a sound-attenuated chamber. An input and output system (photobeam detector, food dispenser, sound card, and house light; Med Associates) was used to control the behavioural training. Rats were rewarded for making a 'go' response (that is, 'hit') within 3 s after target stimulus presentation. Whereas a failure to respond within the 3-s time window after the target stimulus was defined as a 'miss', a go response outside the time window was defined as a 'false alarm'. A go response within 3 s of a non-target stimulus was defined as a 'false positive', and the absence of a response was defined as a 'withhold'. A miss, false alarm, or false positive initiated a 9-s 'time-out' period during which no acoustic stimuli were presented and the house light was turned off. A withhold did not produce a reward or a time out. During the training and testing, trials were grouped into blocks of 50. At the conclusion of each block, a hit ratio (H; number of hits/number of target trials, expressed as a percentage) and a false positive ratio (F; number of false-positives/number of non-target trials, expressed as a percentage) were calculated. The discrimination ability was quantified by the performance score, calculated as H-F×H. ABR measurement and cortical mapping Under pentobarbital anaesthesia (50 mg per kg body weight), ABRs were recorded by placing three electrodes subdermally at the scalp midline, posterior to the stimulated ear, and on the midline of the back 1–2 cm posterior to the neck. Tone pips (4, 8, 16, 20, or 28 kHz) at different intensities were generated using TDT System III (Tucker-Davis Technologies) and delivered to the left ear through a STAX earphone (STAX). The sound intensity that activated a minimal discernable response was defined as the ABR threshold. Cortical responses were recorded with parylene-coated tungsten microelectrodes (1–2 megohms at 1 kHz; FHC). At each recording site, the microelectrode was lowered orthogonally into the cortex to a depth of ~500 μm (layers 4 and 5), where vigorous stimulus-driven responses were recorded. A software package (SigCal, SigGen, and Brainware; Tucker-Davis) was used to calibrate the earphone, generate acoustic stimuli, monitor cortical response properties online, and store data for offline analysis. The overall boundaries of the A1 were functionally determined using non-responsive sites and responsive sites that did not have a well-defined pure tone-evoked response area (that is, non-A1 sites). Overlap index of the tuning curves was computed by first transforming the frequency-tuning curves recorded from two cortical sites into one-dimensional vectors and then calculating the peak of the normalized correlation coefficient between the two vectors produced [31] , [44] . Indices were obtained for all pairs of recording sites with various distances within a single animal. Trains of 6 tonal pulses (25 ms duration with 5 ms ramps at 60 dB SPL) were delivered 4 times at each of 8 repetition rates (2, 4, 7, 10, 12.5, 15, 17.5 and 20 p.p.s.) to document cortical RRTFs. The tone frequency was set at the CF of each site. To reduce the variability resulting from different numbers of neurons included in different multi-unit responses recorded, the normalized cortical response for each repetition rate was calculated as the average response to the last five pulses divided by the response to the first pulse [19] , [25] . The RRTF is the normalized cortical response as a function of the temporal rate. Vector strength [45] , [46] , [47] was calculated using the following equation: where n =total number of spikes, t i ( i =1, 2 ... n) is the time between the onset of the first pulses and the i th spike, and T is the inter-stimulus interval. Spikes that occurred during a 6 T period after the onset of the first tonal pulse were included to compute vector strength. Misclassification rates were calculated by using the Van Rossum spike train distance metric, as described before [26] , [31] . Briefly, each spike train was convolved with an exponential function, N ( t )= N 0 e − t / t , to obtain a filtered function. The distance between two spike trains was defined as the integral of the squared difference of the two functions. Distances were computed for all spike trains at a t of 10 ms for every combination of spike trains in response to pulse trains of various repetition rates. The confusion matrices were constructed by calculating the average distance and s.d. between spike trains in response to stimuli of different or same rates. For spike trains obtained with stimuli of different rates, a misclassification occurred when the distance between the two trains was less than 1 s.d. away from the average distance. For spike trains obtained with stimuli of identical rates, a misclassification occurred when the distance between the two trains was more than 1 s.d. away from the average distance. Recording in silence for 10 periods of 10 s spontaneous neuronal spikes from two-to-four electrodes simultaneously allowed examination of the degree of synchronization between cortical sites. Cross-correlation functions were computed from each electrode pair by counting the number of spike coincidences for time lags of −50 to 50 ms with 1-ms bin size and were normalized by dividing each bin by the square root of the product of the number of discharges in both spike trains [48] . The degree of synchronization was expressed as a percentage of synchronized events. For neural synchrony recording, offline spike sorting, using TDT OpenSorter (Tucker-Davis), was carried out to include only single units in the analysis. Immunohistochemistry Rats received a lethal dose of pentobarbital (85 mg per kg body weight) and were perfused intracardially with saline solution followed by 4% paraformaldehyde in 0.1 M potassium phosphate buffered saline (pH 7.2). Brains were removed and placed in the same fixative containing 20% sucrose for 12–24 h. Fixed material was cut in the coronal plane on a freezing microtome at 40 μm thickness. Free-floating sections were preincubated in a blocking solution to suppress nonspecific binding. The sections were then incubated at 4 °C for 48–72 h in anti-parvalbumin (1:2,000; Sigma) or anti-BDNF (1:300; Millipore). After exposure to biotinylated IgG (1:200; Vector) at room temperature for 1 h, samples were treated with streptavidin-conjugated Cy3 (1:200; Jackson ImmunoResearch) at room temperature for 1 h. Tissues from different rat groups were always processed together during immunostaining procedures to limit variation related to antibody penetration, incubation time, and the post-sectioning condition of the tissue. In anti-PV-free or anti-BDNF-free control experiments, no specific staining was observed in all sections incubated. Fluorescence in the immunostained material was assessed and images were acquired using a Nikon E800 epifluorescent microscope equipped with a camera (AxioCam, Zeiss). A neuron was counted only if the staining revealed a complete soma perimeter and the neuron was clearly differentiated from background. Additional sets of sections from different rat groups were also stained for Nissl substance to determine the cortical laminar boundaries. Statistical analysis Data are presented as means±s.e.m. Unless specified otherwise, statistical significance was assessed using a two-tailed (unpaired) Student's t -test or One-way ANOVA with post-hoc Student-Newman-Keuls test. Significance level was 0.05. How to cite this article: Zhou. X. et al . Environmental noise exposure degrades normal listening processes. Nat. Commun. 3:843 doi: 10.1038/ncomms1849 (2012).